Female monopolization mediates the relationship between pre- and postcopulatory sexual traits Theory predicts a trade-off between investments in precopulatory (ornaments and armaments) and postcopulatory (testes and ejaculates) sexual traits due to the costs associated with their growth and maintenance within the finite energy resources available. Empirical studies, however, have revealed considerable inconsistency in the strength and direction of relationships among these sexual traits. Ambiguity may result from variance in the marginal benefits gained by increasing investments in either pre- or postcopulatory sexual traits. Here, in a broad comparative study, we test the prediction that the relationship between pre- and postcopulatory sexual traits differs among taxa relative to the importance of male–male contest competition within them. We find that covariance between pre- and postcopulatory sexual traits gradually shifts from strongly positive to strongly negative with increasing male–male contest competition. Thus, our findings reveal a potentially unifying explanation for the oftentimes inconsistent relationships in the strength and direction of covariance among sexual traits. Precopulatory sexual selection is one of the primary forces underlying the evolution of extravagant phenotypic structures, including weapons used in male–male combat over access to females and/or male ornaments to attract females [1] , [2] . The bearer’s success in acquiring matings is typically influenced by the size or elaboration of these sexually selected traits [2] . However, since females often mate with multiple males [3] , sexual selection can continue after mating, with sperm from different males competing for fertilization of a female’s ova [4] and/or females biasing the chances of fertilization among competing ejaculates [5] , [6] . Consequently, a male’s overall fitness is determined by his competitiveness during both pre- and postcopulatory selective episodes [7] , [8] . Yet, while these episodes have separately attracted much attention in the study of sexual traits, very little is known about their interaction in explaining patterns of trait evolution. Producing and maintaining weapons used in precopulatory contest competition and ejaculate traits important in postcopulatory sperm competition can be energetically demanding [9] , [10] , [11] , [12] . Consequently, sperm competition models assume that energy allocated to mate acquisition limits investment in ejaculate production, leading to the prediction that investment in testes should trade off against the investment in weaponry used in male–male contest over access to mates [13] . Nevertheless, generating predictions for the direction and strength of the presumed covariance between pre- and postcopulatory traits can be complex. For example, the expression of trade-offs between pre- and postcopulatory traits is likely to depend on the marginal benefits gained by increasing investment in either pre- or postcopulatory sexual traits. To examine how variance in allocation strategies differentially influences the evolution of sexual traits, Parker et al. [13] described the mate-competition loading, a , which refers to the marginal reproductive gains associated with increasing investment in weaponry. Specifically, reproductive gains associated with increased investment in precopulatory weaponry outweigh the added costs of expenditure on weaponry when a >1 (that is, in cases of male–male contest competition rather than scramble competition). Parker et al. [13] then predicted that investment in ejaculates should decrease with any increase in either a or the number of males competing for a given mating. Because of the covariance between a and the number of competing males, pre- and postcopulatory reproductive investments would be expected to trade off when a >1 (contest competition) but not when a ≤1 (scramble competition). Consequently, the relationship between investment in pre- and postcopulatory traits may vary among taxa depending on the relative importance of male–male contest competition for mate monopolization. To date, only few studies have examined the relationship between investments in pre- and postcopulatory sexual traits. Intraspecifically, male investment in weaponry used in male–male competition (for example, horns, large male size relative to females, or grasping forearms) appears to be negatively associated with testes size or ejaculate size in most species examined (for example, dung beetles Onthophagus nigriventris [14] , dung flies Sepsis punctum [15] , myobatrachid frogs Crinia georgiana [13] and freshwater crayfish Austropotamobius italicus [16] ). However, antler size covaries positively with relative testes size and sperm quality in the red deer Cervus elaphus [17] , and relative testes size does not differ between male tree weta Hemideina crassidens exhibiting small and large mandibular weaponry, respectively [18] . Similar inconsistencies are found at the macroevolutionary scale. For example, negative covariance between investment in precopulatory weaponry (in this case the degree of male body size exceeding female size) and either testicular or genital size have been documented across a range of acanthocephalan parasitic worms [19] and pinnipeds (that is, seals, sea lions and walrus) [20] , but no significant relationships were found across onthophagine dung beetles (Coleoptera: Scarabaeidae [14] ) or a wide range of mammals [21] . Finally, across bushcrickets (Orthoptera: Tettigoniidae), the size of the sperm-containing ampulla of spermatophores, and thus ejaculate size, increases with the degree of sexual size dimorphism [22] . The current ambiguity in our understanding of the relationship between pre- and postcopulatory traits represents a major impediment to our understanding of reproductive trait evolution. Comparing the direction of macroevolutionary trends among different taxa can reveal important information on how variance in allocation strategies differentially influences the evolution of sexual traits. However, such a systematic comparison, including an empirical test of Parker et al. ’s [13] prediction, is yet to be done. Here, we studied interspecific associations between pre- and postcopulatory sexual traits in both vertebrate and invertebrate taxa. We then combined our findings with previously published data from additional taxa to test Parker et al. ’s [13] prediction that intra-taxonomic differences in the occurrence of female monopolization influence the covariance between sexual traits important in pre- and postcopulatory sexual selection. Specifically, we assumed that in taxa where males are rarely able to monopolize females, male–male competition before and after mating would be equally important, such that selection would favour both pre- and postcopulatory sexual traits and generate positive covariation between them. By contrast, if female monopolization is very common and thus the mate-competition loading a high within a taxon, investments in precopulatory male–male competition should be more important. Consequently, investments in postcopulatory sexual traits would decrease relative to those in precopulatory traits either through differential allocation or because intense female monopolization would increasingly limit the opportunities for sperm competition (and thus the value of investing in postcopulatory traits). Our overall prediction based on Parker et al. ’s [13] models therefore was that an increasing value of a (or the importance of female monopolization within a taxon) would gradually shift the strength and direction of intra-taxonomic covariation between pre- and postcopulatory sexual traits from strongly positive to strongly negative. In accordance with Parker et al. ’s [13] predictions, we find that the relationship between pre- and postcopulatory sexual traits gradually shifts from strongly positive to strongly negative with increasing male–male contest competition. This dependence on the prevalence of male–male contest competition provides a potentially unifying explanation for why the strength and direction of covariance among sexual traits often varies among studies. Relationships between pre- and postcopulatory sexual traits We collected data on pre- and postcopulatory sexual traits from the literature for seven taxa, including mammals (primates, ungulates), birds (pheasants and allies), fish (minnows), insects (stalk-eyed flies, dung beetles) and schistosomes (blood-flukes). In all these taxa, sexually selected traits important in both selective episodes are well characterized ( Supplementary Note 1 ). Within each taxon, we examined the relationship between the expression of sexually dimorphic traits under precopulatory sexual selection (for example, sexual size dimorphism, the length and dimorphism of canines, size of horns and antlers, tarsal spur length or the span of eye stalks) with interspecific variation in relative testes size (combined testes mass or mean testis length; testes number in schistosomes), a commonly used proxy for the strength of postcopulatory sexual selection [23] , [24] , [25] , [26] . All sexually selected traits are described in the Methods section; for complete data sets and phylogenies see Supplementary Tables 1–6 , Supplementary Figs 1–6 and ref. 27 (for minnows). We first focused our analysis on the relationship between sexual size dimorphism (SSD), a proxy for the strength of precopulatory sexual selection [28] , [29] , [30] , and testes size as a proxy for postcopulatory sexual selection (see above), using phylogenetic multiple regressions controlling for body size (mass or length; Supplementary Note 1 ). Importantly, two previous studies demonstrated that among species of acanthocephalan parasitic worms (Acanthocephala) [19] and pinnipeds [20] , the levels of SSD are inversely related to investment in testicular tissue, showing that the negative covariance between pre- and postcopulatory investment modelled by Parker et al. [13] can be expressed in these traits. However, we found either no, or positive, covariation between precopulatory sexual traits and investment in testicular tissue in our interspecific comparisons, and no evidence of negative relationships between these traits. 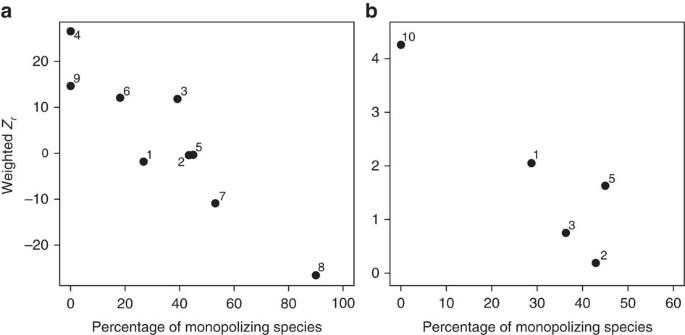Figure 1: Covariation between sexual traits relative to the prevalence of female monopolization. Negative Pearson’s product moment correlation of the taxon-specific weighted effect sizesZrof relationships between testes size and (a) SSD or (b) male weapon size, respectively, against the taxon-specific percentages of species exhibiting female monopolization ((a) Pearson’s product moment correlation,r=−0.92,N=9,P=0.0008; (b) Pearson’s product moment correlation,r=−0.91,N=5,P=0.05). All values of female monopolization are arcsine square-root transformed and then converted to percentages by multiplying by 180/π. For example, testes size increased with SSD in minnows and pheasants and allies, and it tended to increase in schistosomes, albeit not significantly so ( Table 1 ). In contrast, testes size was not correlated with SSD in any other taxon examined (including primates, ungulates and stalk-eyed flies; Table 1 and Supplementary Table 7 ). Table 1 Body-size controlled relationships between testes size and sexual size dimorphism. Full size table Next, we examined the relationship between investment in testes size and weapons (canines, horns, antlers, spurs, eye span) known to influence the outcome of precopulatory male–male contests. These analyses revealed that, after controlling for body size, testes size did not covary significantly with canine length among primates, horn and antler size among ungulates, horn length among dung beetles, tarsal spur length among pheasants and their allies, or eye span among stalk-eyed flies ( Table 2 ). Similarly, in taxa where both males and females express weapons, testes size was not correlated with sexual dimorphism in weapon size ( Supplementary Table 8 ). Table 2 Body-size controlled relationships between testes size and the size of male weaponry. Full size table As Tables 1 and 2 indicate, the phylogenetic scaling parameter λ varied considerably among taxa, with values being comparable between the analyses using SSD and weapon size, respectively. Whereas the reported relationships appeared to be largely independent of the underlying phylogeny in the ungulates, a very strong phylogenetic signal was found in other taxa, such as the pheasants and allies or the schistosomes ( Tables 1 and 2 ). The λ value for the stalk-eyed flies was very small in both cases (<0.0001), but the models were also not significantly different from models with λ set to 1, which is likely to be due to the very small sample size. Despite this variation in λ , however, there was no inter-taxonomic relationship between λ and the intra-taxonomic sample sizes (that is, numbers of species), percentages of female monopolization or weighted Z r values (Pearson’s product moment correlations, all P >0.26). Consequently, our limited data do not currently suggest a link between macroevolutionary patterns and the phylogenetic history of the taxa, and it is beyond the scope of our study to try to understand the role of the phylogenetic signal in the evolution of sexually selected traits. Female monopolization and investment in male sexual traits We tested whether the variable interspecific relationships observed between pre- and postcopulatory traits are influenced by the degree to which competition allows males to monopolize access to females, our proxy for Parker et al. ’s [13] mate competition loading a . To do this, we combined the data presented in Table 1 with additional comparative data sets from the literature, including data on pinnipeds [20] , acanthocephalan parasitic worms [19] and bushcrickets [22] (no additional datasets could be located to expand the results of Table 2 ). On the basis of Parker et al. ’s [13] predictions, we assumed that, across taxa, a would be an increasing function of the proportion of species in each taxonomic group with female monopolization, and that high female monopolization should be associated with increased investment in weaponry and reduced investment in testes size. For each of the taxonomic groups, we thus characterized mating behaviours and territoriality for as many of the species examined in phylogenetic regressions as possible, and considered female monopolization to be present if male–male contest competition influences reproductive success. Specifically, we considered female monopolization to be present in species with female defence polygyny (for example, haremic species), while classifying species with scramble-competition polygyny, resource-defence polygyny, lek polygyny or monogamy to exhibit low or no female monopolization (see Table 3 and Supplementary Note 1 ). We used this approach to determine taxon-specific proportions of species that exhibit female monopolization (see ref. 31 for a similar classification across taxa) and found that the proportion of female monopolization varied widely among the taxonomic groups examined ( Table 3 ). We then converted the effect sizes (partial correlation coefficients r from the multiple regressions between weapons and testes size), which provide a measure of the strength and direction of the association between pre- and postcopulatory traits, to Z r values using Fisher’s transformation weighted by sample size [32] . Table 3 Female monopolization and the relationship between pre- and postcopulatory sexual traits. Full size table In a Pearson’s product moment correlation examining the relationship between weighted effect size values and the proportion of female monopolization (arcsine square-root transformed) across nine taxa, Z r was negatively associated with the taxon-specific percentages of species exhibiting female monopolization (Pearson’s product moment correlation, r =–0.92, N =9, P =0.0008; Fig. 1a ). This negative relationship also remained significant when taxonomic groups with either no monopolization (0%; Pearson’s product moment correlation, r =–0.89, N =7, P =0.008) or complete monopolization (100%; Pearson’s product moment correlation, r =–0.84, N =8, P =0.01) were removed from the analysis. Examining the five vertebrate and four invertebrate taxa separately also yielded negative relationships in both cases, although the association among vertebrates was not statistically significant (vertebrates: Pearson’s product moment correlation, r =–0.80, N =5, P =0.11; invertebrates: Pearson’s product moment correlation, r =–0.99, N =4, P =0.04). Overall, and in accordance with Parker et al. ’s [13] prediction, these results indicate that negative relationships between pre- and postcopulatory traits are more likely in taxonomic groups where female monopolization is common, while positive relationships between pre- and postcopulatory traits occur in groups where female monopolization is either rare or absent. Figure 1: Covariation between sexual traits relative to the prevalence of female monopolization. Negative Pearson’s product moment correlation of the taxon-specific weighted effect sizes Z r of relationships between testes size and ( a ) SSD or ( b ) male weapon size, respectively, against the taxon-specific percentages of species exhibiting female monopolization (( a ) Pearson’s product moment correlation, r =−0.92, N =9, P =0.0008; ( b ) Pearson’s product moment correlation, r =−0.91, N =5, P =0.05). All values of female monopolization are arcsine square-root transformed and then converted to percentages by multiplying by 180/π. Full size image We found similar trends when examining the expression of male weapons instead of sexual dimorphism in body size. Although none of the relationships between pre- and postcopulatory sexual traits were significant among the five taxonomic groups with complete data ( Table 2 ), their weighted Z r values tended to decline with an increasing proportion of species classified as monopolizing females (Pearson’s product moment correlation, r =–0.91, N =5, P =0.05; Fig. 1b ). This result is consistent with the patterns found for SSD, but since the relationship appears to be primarily driven by the dung beetles (data point 10) in our small data set, additional data are clearly needed for a more robust analysis before we can draw more general conclusions. Our results revealed a potentially unifying pattern of relative resource allocation among sexual traits, at least for traits directly involved in pre- and postcopulatory male–male competition. We found that, although the interspecific relationships between pre- and postcopulatory sexual characters appear to be inconsistent among taxonomic groups, the strength and direction of these associations are inversely related to the proportion of species exhibiting female monopolization within each group. These results provide empirical support for Parker et al. ’s [13] theoretical prediction that the importance of female monopolization within a taxonomic group should influence the covariance between sexual traits important in pre- and postcopulatory sexual selection. We found that in taxonomic groups where male contest competition has a strong impact on mate monopolization (for example, pinnipeds), testes size is inversely related to sexual size dimorphism, a premating sexual trait involved in determining access to females. By contrast, these interspecific relationships were positive in taxa where female monopolization is rare or absent. Although limited to only five taxonomic groups and thus with relatively low statistical power, we found a similar pattern for external structures known to be involved in male–male contest competition, with the strength of the interspecific weapon size—testes size relationships tending to decline with increasing percent female monopolization across taxa. Compared with SSD, however, none of the intra-taxonomic relationships were statistically significant. While this may seem somewhat surprising given the assumed expense of these weapons and their importance in mediating postcopulatory sexual selection through female monopolization (see below), it should be noted that all taxa included in this analysis exhibited less than 50% female monopolization. Consequently, it is too early to draw firm conclusions, but the overall similarity to our findings for SSD suggests that the dependence of covariance between sexual traits on female monopolization may be a more general pattern. We thus encourage further intraspecific and/or comparative studies on these links for a broader empirical examination of Parker et al. ’s [13] theoretical predictions. Overall, our data suggest that if male–male contest competition determines access to mates, testes size might be traded against investment in precopulatory sexual traits. Alternatively, postcopulatory sexual selection might simply become increasingly less important as the level of female monopolization increases, being negligible where dominant males can prevent any other male from mating with the females in their harems (that is, complete female monopolization). Therefore, testes size (and possibly other postcopulatory sexual traits) might evolve as a direct function of the intensity of premating sexual selection through male–male contest competition. In fact, similar to our inter-taxonomic comparison, closer examination of the pinnipeds reveals that a negative relationship between testes size and SSD is found among haremic but not among non-haremic species [20] . This result corroborates the findings of the present study within a single taxonomic group by also suggesting that negative covariance between pre- and postcopulatory male investments may be limited to groups of species where male mating success is associated with female monopolization. In other taxa, where female monopolization is less common, mate searching or postcopulatory sexual selection might be more important. However, even if sperm competition is the primary target of sexual selection within a taxonomic group, species exhibiting intense sperm competition are more likely to also show some level of precopulatory male competition (through males’ attempts to avoid sperm competition) than species where selection on male–male competition in general is less intense, which could then result in positive interspecific covariation between pre- and postcopulatory sexual traits. Male–male competition may explain a smaller proportion of the variance in male mating success either because male control over female mating is constrained (for example, external fertilization in minnows) or because sexual selection acts on traits involved in male–male contests as well as traits important for female mate choice (for example, song in bushcrickets [33] or plumage and other sexual traits in pheasants and allies [34] ). These morphological or physiological male ‘ornaments’ can also incur considerable energetic costs (for example, bushcricket song [33] ). By diverting resource allocation away from male contest traits, both pre- and postcopulatory sexual traits associated with male–male competition might be under positive selection (either by concerted or independent evolution), and negative covariance might be found between these traits combined and the expression of male ornaments rather than between the competition traits themselves. These patterns are comparable to previous reports documenting that strong selection for sexually selected traits can generate positive covariance among pre- and postcopulatory traits that combined are negatively related to life-history traits such as somatic maintenance, immunity or longevity [35] , [36] . There is some, albeit indirect, evidence supporting the above hypothesis that competition traits combined might be inversely related to ornaments. A recent study on the macroevolutionary gains and losses of various sexual characters among pheasant species suggests that characters associated with male–male contests tend to show a greater rate of gains than losses, whereas intersexual display traits show the opposite trend [34] . Whether these opposite evolutionary trajectories are the result of trade-offs as opposed to independent evolution and whether similar trends exist in other taxa remains to be seen. Our finding of a dependence of pre- and postcopulatory trait covariance on female monopolization may also extend predictions resulting from resource acquisition-allocation models. These models predict that the sign and strength of between-trait covariance are the result of differences in the mean and variance of resource acquisition relative to resource allocation [37] . Specifically, if males are better at acquiring or defending resources and use them more efficiently, they can afford to invest relatively more in both pre- and postcopulatory reproductive traits than others, resulting in positive trait covariation across males even in the presence of intra-male allocation trade-offs [38] . A good example is presented by stalk-eyed flies, in which the titre of juvenile hormone (JH), a critical regulator of development and metamorphosis in insects, mediates an allocation trade-off between the sexually selected eye stalks and testes within developing males [39] . Despite this intra-male trade-off, the two traits covary positively across males in wild populations [40] , possibly through pleiotropic effects of JH or variation in larval resource acquisition combined with a nutrition-dependent JH titre [41] , [42] . By contrast, a negative association between sexual traits would be expected if males vary little in the total acquired resources but greatly in their allocation to different traits [38] . Although the interaction between resource acquisition and allocation prevents direct inferences about trait covariance at the macroevolutionary scale based on such intraspecific patterns [38] , the general arguments about resource-dependent trait covariance should also apply to higher taxonomic levels [43] . For example, populations or species may differ in their diet type and/or quality, in the abundance and distribution of resources, or in life-history investments (for example, metabolism or survival). These effects may ultimately determine the relative allocation to sexual traits and the potential for selection to act on them [13] , [43] . Whichever the taxonomic level, any biases in resource acquisition and allocation to pre- and postcopulatory male-male competition may not be independent of the level of female monopolization. First, resource allocation may determine the expression of precopulatory contest traits, thereby influencing a male’s ability to prevent rival males from mating with his monopolized females and ultimately determining the degree of postcopulatory sexual selection experienced (and selection on the testes). Second, depending on the importance of female monopolization in explaining male fitness and on which trait has the greatest fitness gain with any marginal increase in size, the acquired resources might be channelled preferentially to either pre- or postcopulatory sexual traits, respectively (see above). Finally, female monopolization might influence resource acquisition itself, with the defence of harems limiting the opportunities to forage and acquire resources for (future) allocation to both pre- and postcopulatory sexual traits. However, to specifically examine such links between resource acquisition-allocation and female monopolization as factors mediating coevolution among sexual traits, more detailed information on the female monopolization capacity than our binary coding of presence/absence would be necessary (for example, mean or maximum harem size and its variance and distribution among species). Although our comparative study has revealed potentially unifying macroevolutionary patterns, detailed intraspecific analyses are needed to understand the basis and adaptive significance of the general evolutionary trends established by such comparative studies (for example, ref. 44 ). Intraspecific analyses are particularly important for discerning relationships among traits due to differences in resource allocation (for example, allocation trade-offs) from other potential sources of covariation among traits (for example, genetic effects, independent selection). To our knowledge, intraspecific data on covariation among pre- and postcopulatory investments relative to female monopolization are currently lacking. It would be interesting to see, however, whether the direction and strength of the intra-population relationship between pre- and postcopulatory traits varies across populations that differ naturally or through experimental manipulation in the intensity of male contest competition. For the purposes of our study, we used relative testes size as a proxy for male investment in sperm production. It should be noted, however, that adaptations to sperm production in response to postcopulatory sexual selection can also involve increases in the density and functional efficiency of the sperm-producing tissue across testes of identical size [45] , [46] , [47] , [48] . Moreover, in addition to sperm competition, selection on testes size can occur through selection against sperm depletion [49] , with males that monopolize more females and thus mate more frequently losing paternity due to sperm depletion [50] . Thus, although the target of selection may be the competitiveness of future ejaculates rather than that of the current ejaculate, similar patterns of investment in sperm production would be expected in both scenarios. Finally, relative testes size can be more intimately linked to premating sexual selection, in that, at least in vertebrates, testes also produce testosterone that can be associated with male aggression and mating success [51] . As a result, testes can be enlarged to primarily increase the output of testosterone, potentially at the expense of considerably less sperm-producing tissue [52] , [53] . Although these different types of selection on testes are unlikely to have any appreciable effect on our key results given the scope of our study, it is important to be aware of such sources of potential unexplained variation when examining the covariance between pre- and postcopulatory sexual traits. In conclusion, we demonstrate that interspecific relationships between pre- and postcopulatory traits are positive in taxonomic groups with rare or no female monopolization but gradually approach zero and ultimately become negative as female monopolization becomes more prevalent within taxonomic groups. These results indicate that intra-taxonomic variance in the strength of female monopolization influences the covariance between sexual traits and reveal important information on how variance in allocation strategies differentially influences the evolution of sexual traits. Data collection and study taxa We collected data on premating weapons, male and female body size, and testes mass or size from the literature for primates, ungulates, pheasants and allies, minnows, stalk-eyed flies, dung beetles and schistosomes ( Supplementary Tables 1–6 ; for data of the minnows exactly as used in our analyses, see ref. 27 ). These taxa exhibit broad variance in the levels of multiple mating, mating systems and mating strategies ( Supplementary Note 1 ). We were not able to account for every taxon-specific difference characterizing the strength of sexual selection, but we considered the variance in the strength of sexual selection within taxa to be more important for the purposes of our study than absolute differences in selection intensity. We focused our analyses on traits that influence male fitness based on intrasexual contests, such as male armaments or sexual size dimorphism, rather than including traits used in female mate choice, for two reasons. First, traits used in female mate choice are extremely diverse, including acoustic, visual, olfactory or behavioural display traits, thereby considerably complicating comparisons across different taxa. In contrast, the diversity in weaponry associated with male contest competition is more readily comparable in terms of resource allocation. Second, studies of the evolution of sexually selected traits tend to be strongly biased towards ornaments and female mate choice, with comparative studies on the evolution of weapons lagging far behind [54] . To calculate sexual size dimorphism (SSD=male size/female size; for example, ref. 55 ), we used body size measured as body mass in all vertebrate taxa except minnows (standard length) and a measure of body length that is widely used for each of the invertebrate taxa except dung beetles (body mass). The use of mass and linear size indices had no effect on the main results ( Supplementary Note 2 ). Note, however, that to avoid the problematic use of ratios in phylogenetic models, we calculated SSD as log(male size/female size), which is equivalent to log(male size)−log(female size). SSD can be biased towards males or females, due to three main processes. First, while selection may favour small males in aerial competition due to higher maneuverability [56] , [57] , the more common contests on the ground typically select for larger males [57] , [58] , [59] , [60] . Second, female-biased SSD can arise through selection on female fecundity, possibly enhanced by male preference for large females [61] , [62] . Third, natural selection may favour different body sizes if dimorphic species can avoid resource competition or increase feeding efficiency by exploiting a wider range of resources compared with sexually monomorphic species [63] , [64] , [65] . In our study, we focused on taxa in which sexual selection is thought to play a critical role in the evolution of SSD in that relatively large males are known to have a mating advantage, and sexual selection is thus likely to act on male size independent of that on female size. This does not entirely reject the possibility that some level of the variation in SSD can be attributed to fecundity selection in females (particularly among insects). Yet, such fecundity selection should not alter our main analysis across taxonomic groups ( Fig. 1 ). First, in the case of fecundity selection, females tend to be larger than males (that is, reversed SSD), but, as sexual selection on male size becomes more intense, the difference between male and female size should decrease. Across species, this would still result in a positive relationship between male/female SSD and the intensity of sexual selection on males, and it is such variance that our analyses captured. Second, we hypothesized that conducting parallel analyses between SSD and weapon size or between vertebrates and invertebrates (that is, where fecundity selection is less or more important, respectively) should control for such confounding effects. Relationships between pre- and postcopulatory sexual traits To assess covariance between pre- and postcopulatory sexual traits while accounting for statistical non-independence of data points by shared ancestry of species, we conducted multiple regressions using phylogenetic generalized least-squared (PGLS) regressions [66] , based on published molecular phylogenies for each taxon ( Supplementary Figs 1–6 , for minnows see ref. 27 ). Using maximum-likelihood methods, these models estimate the phylogenetic scaling parameter λ to evaluate the phylogenetic relationship of the covariance in the residuals [66] . We used likelihood ratio tests to establish whether the models with the maximum-likelihood value of λ differed from models with values of λ =0 or λ =1, respectively, with λ not significantly different from 0 indicating phylogenetic independence and λ not significantly different from 1 indicating a complete phylogenetic association of the traits [66] . Except for the primate phylogeny, branch lengths were unknown. For consistency, we thus assigned equal branch lengths to all phylogenies. In all analyses testing for relationships between pre- and postcopulatory traits, we used testes size as the dependent variable and the precopulatory sexual trait (for example, sexual size dimorphism) as the independent variable and accounted for allometric effects by including male body size as a covariate [67] , [68] . All analyses were performed using the statistical package R version 2.15.2 (ref. 69 ), and all non-normal data distributions were transformed by logarithmic transformations (in the case of pheasant spur length as Y ′=log( Y +0.001) due to zero values) to meet the parametric requirements of the statistical models. Female monopolization and investment in male sexual traits To test Parker et al. ’s [13] predictions on the covariation between investments in pre- and postcopulatory reproductive traits relative to the degree to which competition allows males to monopolize access to females (the mate-competition loading, a ), we evaluated the relationship between the sample-size weighted effect size ( r ) of partial correlation coefficients between pre- and postcopulatory sexual traits derived from our multiple regression models (data taken from Table 1 and published studies [19] , [20] , [22] or from Table 2 , respectively) and the proportion of species within each taxon that exhibit female monopolization ( Table 3 ). Because sample sizes differed among the taxa examined, we converted the r -values listed in Tables 1 or 2 , and calculated from published studies to Z r -values using Fisher’s transformation and weighted them by sample size to obtain a weighted Z r for each taxon [32] . To determine the proportion of species within each taxon that exhibited female monopolization, we characterized mating behaviours and territoriality for as many of the species examined in phylogenetic regressions as possible. Specifically, we focused on categorizing the number of species in which male–male contest competition influences reproductive success within each taxon. These classifications (described in detail in the Supplementary Note 1 ) were applied to all nine taxa for which data on SSD as the premating trait involved in male-male competition were available. We used the proportion of female monopolization in each taxon as a proxy measure for the mate-competition loading factor, a (as defined by ref. 13 ). We examined the relationship between Z r and female monopolization using a linear regression on arcsine square-root transformed monopolization values. Although criticized by Warton and Hui [70] , this transformation was equally successful in improving the residual distribution as the recommended empirical logistic transformation, but it retained a directly interpretable x -axis (that is, 0–100% monopolization), which we rated more important than the slope parameters. Regardless of the transformation (and even without transformation), the effect size of the inter-taxonomic relationship remained identical. Because of the small sample sizes in these analyses, we estimated the P -values using randomization tests (R package lmPerm ) [69] with 1,000 permutations. How to cite this article: Lüpold, S. et al. Female monopolization mediates the relationship between pre- and postcopulatory sexual traits. Nat. Commun. 5:3184 doi: 10.1038/ncomms4184 (2014).